Early life stress in fathers improves behavioural flexibility in their offspring Traumatic experiences in childhood can alter behavioural responses and increase the risk for psychopathologies across life, not only in the exposed individuals but also in their progeny. In some conditions, such experiences can however be beneficial and facilitate the appraisal of adverse environments later in life. Here we expose newborn mice to unpredictable maternal separation combined with unpredictable maternal stress (MSUS) for 2 weeks and assess the impact on behaviour in the offspring when adult. We show that MSUS in male mice favours goal-directed behaviours and behavioural flexibility in the adult offspring. This effect is accompanied by epigenetic changes involving histone post-translational modifications at the mineralocorticoid receptor (MR) gene and decreased MR expression in the hippocampus. Mimicking these changes pharmacologically in vivo reproduces the behavioural phenotype. These findings highlight the beneficial impact that early adverse experiences can have in adulthood, and the implication of epigenetic modes of gene regulation. Adverse environmental conditions in early life can alter stress responses [1] and affect behavioural and cognitive functions in adulthood [2] . Further, they often not only affect the individuals directly exposed to these conditions but also their progeny [3] , [4] . In human, traumatic stress during childhood increases the risk for psychiatric conditions such as borderline personality disorder, bipolar depression, attention deficit hyperactivity disorder and anti-social behaviours across families [5] , [6] . Animal models have also shown that early life stress such as maternal separation or reduced bedding, have negative consequences on behaviour including impaired stress responses, increased behavioural despair and cognitive deficits in adulthood [7] , [8] . However in some cases, early trauma can be beneficial and confer some advantage later in life. In human, mild-to-moderate stressors experienced in childhood can have a ‘stress inoculating’ effect, and favour adaptive responses and resilience upon exposure to other stressors later in life [9] , [10] . Likewise in animals, chronic exposure to adverse conditions in postnatal life can in some conditions lower stress reactivity and improve cognitive abilities like spatial and reversal learning in adulthood [11] , [12] . Whether such beneficial effects can also be observed in the offspring has however not been investigated. Using a model of unpredictable maternal separation and maternal stress (MSUS) in mice [13] , we examined whether trauma exposure in postnatal life can have beneficial effects on behaviour in the offspring. This model aims at mimicking real-life conditions in humans that can occur in disrupted families with unpredictable and unreliable parental care, parental neglect and disorganized and poor affective attachment. We found that MSUS favours goal-directed behaviours and reversal learning in the offspring, suggesting an effect on behavioural flexibility. This is accompanied by epigenetic changes at the mineralocorticoid receptor (MR) gene and decreased MR expression, that can be mimicked in vivo by pharmacological blockade of MR. These findings highlight the potential adaptive benefit of adverse experiences in early life, and implicate a stress hormone receptor and its epigenetic regulation. The impact of MSUS on goal-directed behaviour We used MSUS [13] to examine whether traumatic stress in postnatal life can have behavioural benefits in the offspring of mice. Second-generation (F2) offspring were obtained by breeding males, subjected to MSUS when pups or control males (F1), to wild-type C57BL/6 adult females ( Supplementary Fig. 1 ). The effect of MSUS on behaviour was first examined using an elevated plus maze (EPM). This maze assesses approach/avoidance, and an animal’s response to risk and potential danger in aversive conditions [14] , [15] . 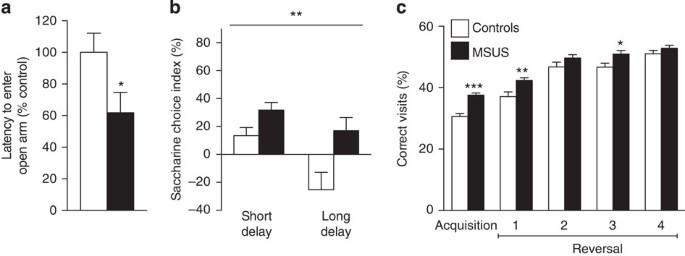Figure 1: Altered behavioural responses in F2 females. (a) Latency to first enter an open arm on the elevated plus maze (controlsn=16, MSUSn=15;t(29)=2.15; Student’s two-tailedt-test). The results were replicated in two independent experiments. (b) Saccharine choice index in the DDT after short (0.5–7 s) or long (7,5 s) delays (controlsn=12, MSUSn=16; F(1,26)=8.21; repeated measures analysis of variance (ANOVA)). Data were collected continuously during 16 consecutive testing days in one experiment. (c) Per cent of correct visits during acquisition and across the first four sessions of reversal on BST (controlsn=13, MSUSn=16; F(1,27)=8.05; repeated measures ANOVA). Data were collected continuously during 26 consecutive testing days in one experiment. Data are represented as mean±s.e.m. *P<0.05, **P<0.01, ***P<0.001. While control males (F1) and females (F2) had a long latency to first enter an open arm, MSUS animals (F1 males and F2 females) had a short latency ( Figs 1a and 2a , Supplementary Table 1 ), indicating reduced aversion and avoidance. Since such behaviour may reflect altered goal-directed and motivated behaviour, we next examined the animals’ response in non-aversive conditions using a delay-discounting task (DDT) in IntelliCages [16] (females were used because Intellicages are not appropriate for males due to interference with social hierarchy resulting from group housing). This task assesses an animal’s choice between a non-appealing but immediate reward (water) and an appealing but delayed reward (saccharine) based on a choice strategy. It also assesses impulsivity. While F2 control females preferentially chose water and minimally delayed their choice for saccharine, F2 MSUS females delayed their choice in favour of saccharine ( Fig. 1b ), suggesting improved goal-directed behaviours. This choice was not due to an increased preference for saccharine since saccharine consumption was similar in control and MSUS animals in normal conditions ( Supplementary Fig. 2 ). Because goal-directed behaviours depend on behavioural flexibility, in particular when rules change during a task [17] , we next tested the animals on a behavioural sequencing task (BST) using IntelliCages, a task assessing response flexibility. For BST, each animal is first trained to alternatively visit two opposite diagonal corners of an arena to obtain a drink reward. Corners assignment is then switched (reversal) to the other diagonal, and the animal has to shift shuttling from corners in one diagonal to corners in the other diagonal while maintaining a goal-directed strategy. On this test, F2 MSUS females made more visits to the correct corners during both, the acquisition and the reversal phase ( Fig. 1c ), suggesting improved flexibility and better adaptation to new rules. We confirmed this effect in males using a differential reinforcement of lower rates (DRL) paradigm, a comparable task that can be used in individual animals and does not require group housing. On the DRL task, an animal can obtain a reward by nose-poking in a hole in response to a cue light after a predefined delay (the cue light signals that the required delay has elapsed). With a 6-sec delay, an easy requirement [18] , F1 control and MSUS males nose-poked a similar number of times at the right delay, indicating proper response ( Fig. 2b ). However, with an 18-second delay, a more demanding requirement, both F1 and F2 MSUS males poked significantly more often than their respective controls at the right delay, indicating better goal-directed behaviours ( Fig. 2c , Supplementary Fig. 3a ). Further, during extinction, nose-poke response was more rapidly extinguished in F1 and F2 MSUS males than in controls ( Fig. 2d , Supplementary Fig. 3b ), suggesting less perseveration. In both F1 males and F2 females, the improved behavioural flexibility was not due to altered learning since response in an active avoidance test was similar in control and MSUS animals ( Supplementary Fig. 4 ). Figure 1: Altered behavioural responses in F2 females. ( a ) Latency to first enter an open arm on the elevated plus maze (controls n =16, MSUS n =15; t (29)=2.15; Student’s two-tailed t -test). The results were replicated in two independent experiments. ( b ) Saccharine choice index in the DDT after short (0.5–7 s) or long (7,5 s) delays (controls n =12, MSUS n =16; F(1,26)=8.21; repeated measures analysis of variance (ANOVA)). Data were collected continuously during 16 consecutive testing days in one experiment. ( c ) Per cent of correct visits during acquisition and across the first four sessions of reversal on BST (controls n =13, MSUS n =16; F(1,27)=8.05; repeated measures ANOVA). Data were collected continuously during 26 consecutive testing days in one experiment. Data are represented as mean±s.e.m. * P <0.05, ** P <0.01, *** P <0.001. 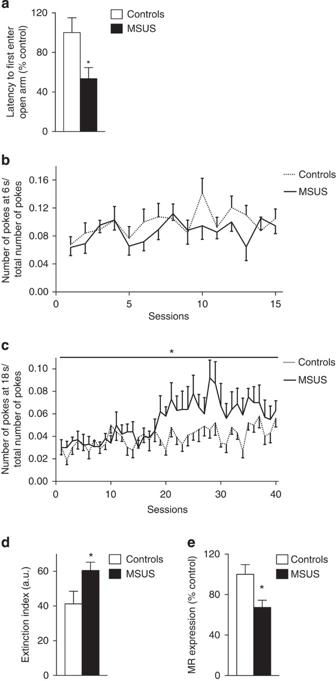Figure 2: Effect of MSUS on goal-directed behaviours and behavioural flexibility andMRexpression F1 males. (a) Latency to first enter an open arm on an elevated plus maze (controlsn=8, MSUSn=18;t(24)=0.79; Student’s two-tailedt-test). Data are representative of three independent experiments. (b) Number of nose pokes after the required delay (6 s) over the total number of pokes on the DRL task (controlsn=12, MSUSn=11; F(1,21)=1.05; repeated measures analysis of variance (ANOVA)). (c) Number of nose pokes after the required delay (18 s) over the total number of pokes on the DRL task (controlsn=11, MSUSn=11; F(1,20)=4.99; repeated measures ANOVA). (d) Extinction index during extinction training on the DRL task (controlsn=9, MSUSn=9;t(16)=−2.19; Student’s two-tailedt-test). DRL and extinction data were obtained daily for 30 min in one 58-day experiment. (e) Quantitative RT–PCR showingMRexpression in the hippocampus in F1 MSUS males (controlsn=7, MSUSn=8;t(13)=2.21; Student’s two-tailedt-test). Data were obtained in two independent experiments. Data are represented as mean±s.e.m. *P<0.05. Full size image Figure 2: Effect of MSUS on goal-directed behaviours and behavioural flexibility and MR expression F1 males. ( a ) Latency to first enter an open arm on an elevated plus maze (controls n =8, MSUS n =18; t (24)=0.79; Student’s two-tailed t -test). Data are representative of three independent experiments. ( b ) Number of nose pokes after the required delay (6 s) over the total number of pokes on the DRL task (controls n =12, MSUS n =11; F(1,21)=1.05; repeated measures analysis of variance (ANOVA)). ( c ) Number of nose pokes after the required delay (18 s) over the total number of pokes on the DRL task (controls n =11, MSUS n =11; F(1,20)=4.99; repeated measures ANOVA). ( d ) Extinction index during extinction training on the DRL task (controls n =9, MSUS n =9; t (16)=−2.19; Student’s two-tailed t -test). DRL and extinction data were obtained daily for 30 min in one 58-day experiment. ( e ) Quantitative RT–PCR showing MR expression in the hippocampus in F1 MSUS males (controls n =7, MSUS n =8; t (13)=2.21; Student’s two-tailed t -test). Data were obtained in two independent experiments. Data are represented as mean±s.e.m. * P <0.05. Full size image The effect of MSUS on the HPA axis Previous studies have implicated components of the hypothalamic–pituitary–adrenal (HPA) axis and their epigenetic regulation in the effects of early stress on behaviour [13] , [19] . We measured the level of corticosterone in serum and observed that it was similar in F2 control and MSUS animals ( Supplementary Fig. 5 ). We also examined whether MR, a mineralocorticoid receptor recently implicated in goal-directed behaviours [20] and in the appraisal of novel environments [21] , is associated with the effects of MSUS. Real-time quantitative reverse transcriptase PCR (RT–PCR) and Western blot analyses showed that MR mRNA ( Fig. 3a ) and protein ( Fig. 3b , Supplementary Fig. 9 ) were significantly lower in the hippocampus of F2 MSUS females, a brain structure involved in adaptive learning and behavioural control [22] , compared with controls. This decrease was also observed in F1 fathers ( Fig. 2e ) and F1 female siblings ( Fig. 3c ), suggesting a consistent downregulation across generations and sex. MR expression was not altered in the olfactory bulb, a brain region unrelated to behavioural flexibility ( Supplementary Fig. 6 ). 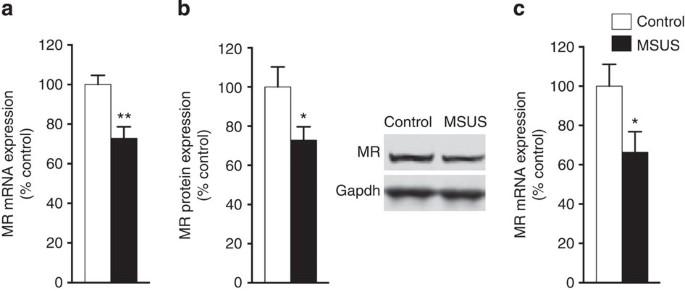Figure 3: Expression analyses ofMRgene. (a) Level ofMRmRNA in the hippocampus of F2 females measured by quantitative RT–PCR (controls=12, MSUSn=7;t(17)=3.54; Student’s two-tailedt-test). These results were reproduced in two independent experiments. (b) Western blot showing MR protein expression in the hippocampus of F2 females (controlsn=7, MSUSn=7;t(12)=2.20; Student’s two-tailedt-test). (c) Level of MR mRNA in the hippocampus of F1 females (controlsn=9, MSUSn=7;t(14)=2.57; Student’s two-tailedt-test). Data are represented as mean±s.e.m; *P<0.05, **P<0.01. Figure 3: Expression analyses of MR gene. ( a ) Level of MR mRNA in the hippocampus of F2 females measured by quantitative RT–PCR (controls=12, MSUS n =7; t (17)=3.54; Student’s two-tailed t -test). These results were reproduced in two independent experiments. ( b ) Western blot showing MR protein expression in the hippocampus of F2 females (controls n =7, MSUS n =7; t (12)=2.20; Student’s two-tailed t -test). ( c ) Level of MR mRNA in the hippocampus of F1 females (controls n =9, MSUS n =7; t (14)=2.57; Student’s two-tailed t -test). Data are represented as mean±s.e.m; * P <0.05, ** P <0.01. Full size image Epigenetic alterations in the MR gene Gene regulation induced by environmental factors implicates epigenetic processes. We therefore examined DNA methylation, an important epigenetic mark for gene regulation, in the MR gene. Quantitative bisulphite pyrosequencing showed that DNA methylation in a region upstream of the transcription start site important for transcriptional regulation [23] ( Fig. 4d ) was similar in the hippocampus of F1 male ( Fig. 4a ) and F2 female ( Fig. 4b ) control and MSUS mice. We then examined histone post-translational modifications (HPTMs), another important epigenetic mark known to be influenced by stress [19] , [24] and associated with transcriptional regulation in the adult mouse hippocampus [25] . Chromatin immunoprecipitation (ChIP) assays showed that acetylation of H4K5 (H4K5ac) and H3K14 (H3K14ac), dimethylation of H3K4 (H3K4me2), and trimethylation of H3K36 (H3K36me3) were significantly decreased at an intragenic region of the MR gene in F2 MSUS hippocampus, while H3K9 (H3K9me2) and H3K27 (H2K27me2) dimethylation were not altered ( Fig. 4c,d Supplementary Table 2 ). The decrease was specific to MR and was not observed at the glucocorticoid receptor ( GR ) gene ( Fig. 5a , Supplementary Table 2 ), consistent with the lack of change in GR expression ( Fig. 5b ). We confirmed that HPTMs alteration in F2 hippocampus is relevant for MR expression by mimicking the decreased acetylation and methylation pharmacologically in vivo . Injection of inhibitors of histone acetyl- and methyl-transferases (C646 and 3-deazaneplanocin A), known to block histone acetylation and methylation in the brain [26] , decreased MR expression in the adult hippocampus ( Fig. 6a ) but did not affect GR expression ( Fig. 6b ). 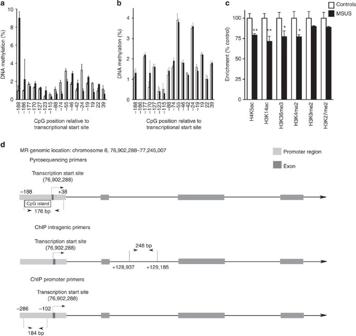Figure 4: Epigenetic analyses ofMRgene. Per cent methylated cytosines for each CpG at theMRpromoter in the hippocampus of (a) F1 males (controlsn=6, MSUSn=5; F(1,9)=0.1; repeated measures analysis of variance (ANOVA)) and (b) F2 females (controlsn=6, MSUSn=7; F(1,11)=0.56; repeated measures ANOVA). Numbers below thex-axis indicate CpG site position. (c) ChIP assays showing H4K5ac (controlsn=6, MSUSn=6;t(10)=6.21; Student’s two-tailedt-test), H3K14ac (controlsn=6, MSUSn=6;t(10)=3.36; Student’s two-tailedt-test), H3K36me3 (controlsn=5, MSUSn=6;t(8)=2.25; Student’s two-tailedt-test), H3K4me2 (controlsn=6, MSUSn=5,t(9)=2.43; Student’s two-tailedt-test), H3K9me2 (controlsn=4, MSUSn=4,t(6)=−1.2; Student’s two-tailedt-test) and H3K27me2 (controlsn=4, MSUSn=4,t(6)=−1.198; Student’s two-tailedt-test) in the hippocampus of F2 females. (d) Genomic location of primers on MR sequence. Pyrosequencing primers located within the CpG island upstream of the transcriptional start site in the promoter region, ChIP primer covering an intragenic region between exon 2 and 3 and ChIP primers covering the promoter region. Primers are indicated as black arrowheads below the sequence. Data are represented as mean±s.e.m.*P≤0.05, **P<0.01. Figure 4: Epigenetic analyses of MR gene. Per cent methylated cytosines for each CpG at the MR promoter in the hippocampus of ( a ) F1 males (controls n =6, MSUS n =5; F(1,9)=0.1; repeated measures analysis of variance (ANOVA)) and ( b ) F2 females (controls n =6, MSUS n =7; F(1,11)=0.56; repeated measures ANOVA). Numbers below the x -axis indicate CpG site position. ( c ) ChIP assays showing H4K5ac (controls n =6, MSUS n =6; t (10)=6.21; Student’s two-tailed t -test), H3K14ac (controls n =6, MSUS n =6; t (10)=3.36; Student’s two-tailed t -test), H3K36me3 (controls n =5, MSUS n =6; t (8)=2.25; Student’s two-tailed t -test), H3K4me2 (controls n =6, MSUS n =5, t (9)=2.43; Student’s two-tailed t -test), H3K9me2 (controls n =4, MSUS n =4, t (6)=−1.2; Student’s two-tailed t -test) and H3K27me2 (controls n =4, MSUS n =4, t (6)=−1.198; Student’s two-tailed t -test) in the hippocampus of F2 females. ( d ) Genomic location of primers on MR sequence. Pyrosequencing primers located within the CpG island upstream of the transcriptional start site in the promoter region, ChIP primer covering an intragenic region between exon 2 and 3 and ChIP primers covering the promoter region. Primers are indicated as black arrowheads below the sequence. Data are represented as mean±s.e.m. * P ≤0.05, ** P <0.01. 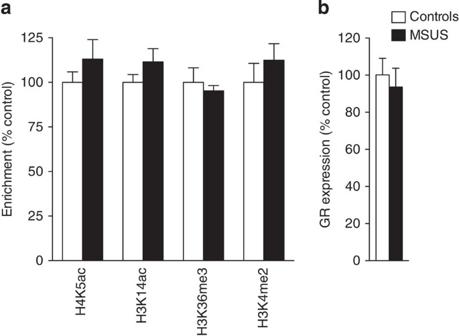Figure 5: Epigenetic and expression analyses ofGRgene. (a) ChIP assays showing histone PTMs at the GR gene in the hippocampus in F2 females (H4K5ac (controlsn=4, MSUSn=4;t(6)=−1.05), H3K14ac (controlsn=6, MSUSn=6;t(6)=−1.33), H3K36me3 (controlsn=4, MSUSn=4;t(3)=0.66) and H3K4me2 (controlsn=6, MSUSn=5;t(3)=−0.86). (b) Quantitative RT–PCR showing GR expression in the hippocampus of F2 MSUS females (controlsn=7, MSUSn=6;t(11)=0.48). Student’s two-tailedt-test was used for all analyses. Data are represented as mean±s.e.m. Full size image Figure 5: Epigenetic and expression analyses of GR gene. ( a ) ChIP assays showing histone PTMs at the GR gene in the hippocampus in F2 females (H4K5ac (controls n =4, MSUS n =4; t (6)=−1.05), H3K14ac (controls n =6, MSUS n =6; t (6)=−1.33), H3K36me3 (controls n =4, MSUS n =4; t (3)=0.66) and H3K4me2 (controls n =6, MSUS n =5; t (3)=−0.86). ( b ) Quantitative RT–PCR showing GR expression in the hippocampus of F2 MSUS females (controls n =7, MSUS n =6; t (11)=0.48). Student’s two-tailed t -test was used for all analyses. Data are represented as mean±s.e.m. 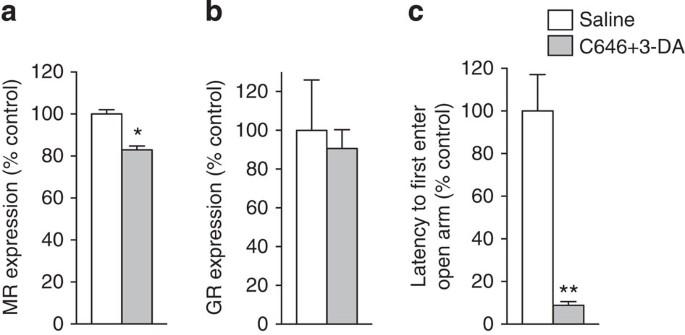Figure 6: Effect of the histone acetyl- and methyl-transferases inhibitors—C646 and 3-DA injection. (a)MRmRNA level (salinen=4, C646+3-DAn=5;t(4.85)=6.47), (b)GRmRNA level (salinen=4, C646+3-DAn=5;t(6)=0.25) and (c) latency to first enter an open arm on the elevated plus maze (salinen=8, C646+3-DAn=9;t(23,6)=5.31) in females. Student’s two-tailedt-test was used for all analyses. Data are represented as mean±s.e.m. *P≤0.05, **P<0.01. Full size image Figure 6: Effect of the histone acetyl- and methyl-transferases inhibitors—C646 and 3-DA injection. ( a ) MR mRNA level (saline n =4, C646+3-DA n =5; t (4.85)=6.47), ( b ) GR mRNA level (saline n =4, C646+3-DA n =5; t (6)=0.25) and ( c ) latency to first enter an open arm on the elevated plus maze (saline n =8, C646+3-DA n =9; t (23,6)=5.31) in females. Student’s two-tailed t -test was used for all analyses. Data are represented as mean±s.e.m. * P ≤0.05, ** P <0.01. Full size image Implication of MR in goal-directed behaviours To examine the link between altered MR expression and behaviour, we tested the effect of HPTMs inhibitors in vivo . Adult females injected with the inhibitors had a decreased latency to first enter an open arm on the EPM, similar to MSUS mice ( Fig. 6c and Supplementary Table 1 ). Likewise, blockade of MR receptor by chronic injection of the competitive antagonist spironolactone decreased the latency to first enter an open arm on the EPM ( Fig. 7b and Supplementary Table 1 ). Real-time quantitative RT–PCR also showed that spironolactone significantly decreased MR expression but did not affect GR expression ( Fig. 7a ). The effect of the drugs on behaviour was not due to increased activity or anxiety since total distance covered on the EPM and time spent in the open arms were not altered by the inhibitors ( Supplementary Fig. 7 ) or by spironolactone ( Supplementary Fig. 8 ). These results therefore strongly suggest a relationship between MR expression and behavioural alterations induced by MSUS. 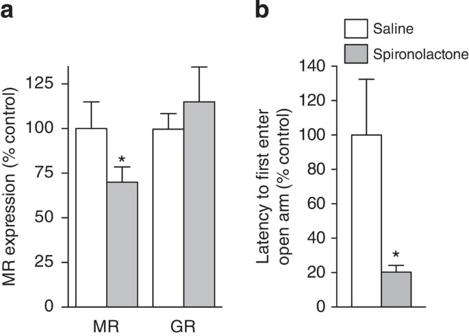Figure 7: Effect of spironolactone injection. (a)MR(t(21)=2.03) andGR(t(21)=0.85) mRNA level (salinen=8, spironolactonen=9; Student’s two-tailedt-test) and (b) latency to first enter an open arm on the elevated plus maze (salinen=8, spironolactonen=9;t(7,21)=2.44; Student’s two-tailedt-test) in adult females. Data are represented as mean±s.e.m. *P≤0.05. Figure 7: Effect of spironolactone injection. ( a ) MR ( t (21)=2.03) and GR ( t (21)=0.85) mRNA level (saline n =8, spironolactone n =9; Student’s two-tailed t -test) and ( b ) latency to first enter an open arm on the elevated plus maze (saline n =8, spironolactone n =9; t (7,21)=2.44; Student’s two-tailed t -test) in adult females. Data are represented as mean±s.e.m. * P ≤0.05. Full size image Assessment of DNA methylation in sperm Since DNA methylation in germ cells has been implicated in epigenetic inheritance [13] , [27] , [28] , [29] , [30] , [31] , we examined the profile of DNA methylation at the MR promoter in the sperm of adult F1 males. Bisulphite pyrosequencing revealed that DNA methylation was significantly increased at several CpGs across the MR promoter ( Fig. 8 ), suggesting a potential implication in the transmission of MR alteration. 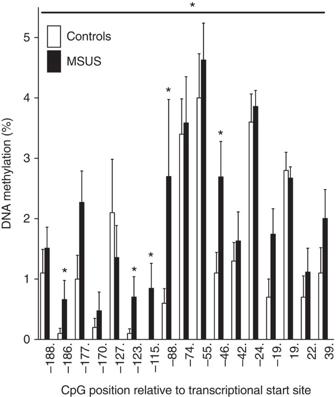Figure 8: DNA methylation at MR promoter in sperm of F1 males. Per cent methylated cytosines for each CpG at MR promoter (controlsn=11, MSUSn=6; F(1,15)=6.77; repeated measures analysis of variance). Numbers below thex-axis indicate CpG site position. Data are represented as mean±s.e.m. *P≤0.05. Figure 8: DNA methylation at MR promoter in sperm of F1 males. Per cent methylated cytosines for each CpG at MR promoter (controls n =11, MSUS n =6; F(1,15)=6.77; repeated measures analysis of variance). Numbers below the x -axis indicate CpG site position. Data are represented as mean±s.e.m. * P ≤0.05. Full size image Experimental paradigms in animal models have reported that early life stress can have different consequences on behaviour, stress reactivity and cognitive performance later in life [32] . Maternal separation during postnatal life in mice or rats for instance, can increase stress reactivity, induce behavioural despair and alter cognitive functions in some models [1] , [7] , [8] , [33] , [34] , [35] , [36] but can have opposite effects in other models [37] , [38] . Although paradoxical at first sight, these findings indicate that the impact of early stress can vary, probably due to differences in experimental paradigms or in the sensitivity of the models. In this respect, our MSUS paradigm is a robust and reliable manipulation that differs from classical models of early life stress such as daily maternal separation or limited bedding [39] , in that it is unpredictable and combines maternal separation with additional maternal stress [13] , [31] , [40] , [41] . The unpredictability prevents overcompensation by extra maternal care and more closely reproduces real-life conditions of traumatic events in humans occurring in abandonment, parental neglect and with violent or abusive parents/caretakers. Our previous work has shown that MSUS induces a range of symptoms including depressive-like behaviours, deficits in social interaction, loss of behavioural control and impaired memory [13] , [40] , [41] , [42] . MSUS is overall more severe than other manipulations when considered in the context of the inverted U-curve model of stress [1] . It negatively affects multiple forms of behaviour, and its effects are transmitted across generations. But at the same time, the behavioural flexibility it induces in challenging situations reflects another programming effect that in contrast, is positive. This corroborates the mismatch hypothesis proposing that early adversity can elicit adaptive responses allowing an individual to better cope with further adversity later in life [11] , [43] . But it also decisively extends this hypothesis by introducing a heritable component to the model. The consequences of early adversity can hence not be generally categorized as negative or positive depending on the severity of stress, but need to be considered in different contexts for each trait depending on the conditions and the situation. We suggest that other models of early life stress may similarly induce opposite effects, that could be revealed using different testing conditions. The data provide novel evidence for the involvement of MR in the impact of early traumatic stress. MR expression and histone acetylation/methylation at the MR gene are reduced by MSUS in the adult hippocampus. Blocking MR activity or inhibiting histone acetyl- and methyl-transferases can mimic MR downregulation and reproduces some of the behavioural symptoms induced by MSUS. While a neurodevelopmental effect cannot be ruled out, these findings strengthen the hypothesis that MR is implicated in goal-directed behaviours and responses to challenge [20] , [21] . Finally, although MR plays an important role, other genes (but not GR ) may also be involved since MSUS is a global manipulation that likely affects multiple pathways. Our results show that, unlike histone PTMs, DNA methylation at the MR gene is not altered by MSUS in the adult hippocampus. The dissociation between a change in histone PTMs and normal DNA methylation suggests that, although interconnected, these epigenetic marks are independent at the MR gene. Nonetheless, in male germ cells, DNA methylation was significantly increased at the MR gene. Previous observations of DNA hypo- and hyper-methylation at loci such as corticotropin-releasing factor receptor 2 and methyl CpG binding protein 2 genes in MSUS male germ cells [13] have suggested the implication of DNA methylation in the transmission of the effects of MSUS across generations. However, in the case of MR, other epigenetic mechanisms such as histone PTMs in sperm may also be involved in transmission. For instance, H3K4me2 can be retained at the MR promoter even after most histones are replaced by protamines during spermatogenesis [44] , and may therefore be transmitted to the offspring. Further, non-coding RNAs in sperm cells have also recently been implicated in the transmission of the MSUS phenotype [42] . Finally, the findings are highly relevant to the clinic because MR is linked to stress-induced pathologies like depression in humans [45] , [46] . They may therefore open novel perspectives for potential use for therapeutic treatment in the future. Animals Adult (3–6-month-old) C57BL/6 mice (Janvier SAS, Berthevin, France) were used. The mice were maintained under a reverse light–dark cycle (light off at 0800 hours) in a temperature- and humidity-controlled facility with food and water ad libitum . Behavioural testing was conducted during the first 5 h of the animals’ active cycle. Both females and males were used for behavioural testing and molecular experiments. All experiments were conducted in accordance with guidelines and regulations of the cantonal veterinary office of Zürich; Licence Nr 55/2012. Treatment For MSUS, dams and litters were subjected to 3-h proximal separation daily from postnatal day 1 to 14. During separation, dams were exposed to either 20-min restraint stress or 5-min forced swim stress unpredictably. Control animals were left undisturbed except for a cage change once a week. Once weaned (postnatal day 21), pups were reared in social groups (4–5 mice per cage) composed of animals of the same sex subjected to the same treatment but from different mothers to avoid litter effects. To obtain second-generation animals, F1 control and MSUS males were mated to naïve primiparous C57BL/6 adult females. Males were removed immediately after mating and were never in contact with their progeny. A total of 30 females (F0, 15 controls and 15 MSUS) were used to generate F1 animals and 54 F1 males (27 controls and 27 MSUS) were used to produce F2 animals in three independent experiments, yielding 14 control and 20 MSUS litters (see Supplementary Fig. 1 for MSUS paradigm). Behavioural testing Behavioural testing was carried out by experimenters blinded to treatment. Behaviours were monitored by direct observation and by automated videotracking (Viewpoint, France). Females were tested in IntelliCages (DDT then BST, 9 weeks in total) and males on the EPM, DRL and active avoidance. For IntelliCages, behaviour was automatically recorded for 1 h twice a day (1100–1200 hours and 1600–1700 hours) in every animal through implanted transponders. Females (2 months old) were implanted with transponders (DATAMARS SA, Bedano/Lugano, Switzerland) under 5% isoflurane anaesthesia to allow individual identification and monitoring. Following implantation, the animals were housed in standard home cages for 1 week then transferred to an IntelliCage in groups of 16 per cage. The IntelliCage (NewBehavior AG, Zürich, Switzerland) is an automated testing device (20 cm height, 55 cm length and 38 cm width) with four conditioning corners. Each corner gives access to two bottles of liquid (one of water and one of 0.5% saccharine solution) through a hole (13 mm; one bottle on each side of the hole). Each hole can be closed with an automated door to prevent access to bottles. The number and duration of nose pokes are recorded by photobeams on both sides of each corner and drinking behaviour is measured by lickometers. Access to water was limited (see protocol below), and food was available ad libitum in a food topper. Females were habituated to an IntelliCage for 7 days during which they had free access to water in each corner. Females that did not adapt to the IntelliCage (no drinking for at least 36 h during habituation) were removed from the cage and excluded from testing. For training on the DDT [47] , all doors were opened and females had free access to water and saccharine in each corner (0 s delay). DDT started when preference to saccharine was established (>50% saccharine licks over all licks). Upon every corner visit, doors giving access to water were always open but doors giving access to saccharine were opened only after a delay (test phase). Doors opening was progressively delayed by an additional 0.5 s each day until the animals shifted their preference to water (<50% saccharine licks over all licks). At the end of training, doors giving access to water and saccharine were then re-opened with no delay for 3 days to confirm the preference of saccharine. For the BST [48] , animals had access to drinking bottles for 1 h per day twice a day (1100–1200 hours and 1600–1700 hours) for 7 days (doors were closed the rest of the time). For acquisition, each animal learned to alternatively visit two diagonal corners of the IntelliCage to collect water (random assignment of diagonal corners for each animal). Re-entry to the same corner or visit to a corner of the other diagonal was not rewarded. Acquisition was followed by eight sessions of reversal after corner assignment was switched to the other diagonal. Reversal was repeated three times. Body weight was measured weekly. The (i) number and duration of visits to each corner (exploratory activity), (ii) number, duration and side (right or left) of nose pokes, (iii) number, duration and side of licks, and duration and side of contacts between the mouse tongue and the bottle spout (considered as index of fluid consumption) were measured. For DDT, preference for saccharine was evaluated by calculating a preference index (100 × ( S − W )/( S + W ) with S =average lick contact time per saccharin choice, W =average lick contact time per water choice (100=consumption of saccharin only). For BST, the percentage of correct visits over total visits per test session was calculated to assess learning. The EPM consisted of two open (no wall) and two closed (with walls) arms (dark grey polyvinyl chloride, 30 cm length, 5 cm width) linked to a central platform and elevated 60 cm above the ground. Each mouse was placed on the central platform facing a closed arm, and allowed to explore the maze for 5 min. The latency to first enter an open arm, the time spent on each arm and total distance covered were automatically recorded by a videotracking system. Experiments were carried out in red light (15 W). For the DRL task, animals had restricted water access for 1 day prior to testing. Four identical operant conditioning chambers (15.9 cm height, 16.5 cm length and 17.5 cm width) with a stainless-steel grid floor (TSE Systems, Germany) were placed in sound-insulated boxes. Each chamber was equipped with a nose-poke response unit (2 cm diameter) fitted with a photocell sensor and a yellow cue light in the hole. A green cue light was located on the wall of the chamber above the nose-poke module. A regular light (2.8 W) located on the ceiling of the box was turned on to signal start and end of each testing session. A liquid dispenser fitted with a photocell sensor was located left to the nose-poke module. Each mouse was habituated to the chamber for 30 min, during which 10 μl of water were delivered to the liquid dispenser every 30 s. The animals were then trained on a continuous reinforcement (CRF) schedule once daily, for which they had to nose-poke for the delivery of 10 μl water during 30-min sessions until they reached a criterion of 50 nose pokes per session. Following CRF, the animals were trained on a DRL phase. During this phase, nose pokes were rewarded only if enough time (defined by a criterion: 6 or 18 s) had elapsed between two consecutive nose pokes. The timer was reset after each reward delivery. Nose pokes done too early (or too late) were not rewarded and reset the timer. A green cue light signalled when a nose-poke could have been rewarded. Each correct nose-poke turned on a yellow light as confirmation. The animals were first tested with a criterion time of 6 s for 3 consecutive weeks (15 testing days) then with a criterion of 18 s for 8 weeks (40 testing days). Testing was followed by 3 days of extinction during which the protocol was the same but the animals were not rewarded. The timing of each nose-poke was recorded by a photocell sensor (±1 s accuracy). Data analyses were conducted in Matlab. The distribution of inter-response time (IRT), which represents the interval between two successive nose pokes, was calculated for each session. IRTs were normalized by dividing the number of IRTs of >1 s by the total number of IRTs. Extinction index is the difference in number of nose pokes before extinction (last 3 days of training) and the third day of extinction. Body weight was measured weekly. Active avoidance was tested using the same operant conditioning chambers as for DRL. Each chamber was equipped with a shock grid floor, and a nose-poke module fitted with a photocell sensor was placed on the left side of one of the chamber walls. A green cue light was located above the nose-poke module. A regular light (2.8 W) located on the ceiling of the box was turned on to signal the start and end of each testing session. Males were habituated to the chamber for 30 min during which the nose-poke module was closed. Two days after habituation, each male was trained to escape from a foot-shock (0.3 mA, max 10 s) by nose-poking over 60 trials for 30 min (one trial every 30 s). If the animal did not nose-poke, the foot-shock was automatically terminated after 10 s. During training, a normal light was always on, a green light was on when there was no shock and a red light was on during shocks. The sensor located in the nose-poke hole recorded the time of occurrence of each nose poke (1 s resolution). Latency to escape and number of escapes were measured and then analyzed in blocks of five trials. Serum corticosterone assay Blood was collected from tail artery after clipping the tail tip then stored at 4 °C over night for coagulation and then centrifuged at 3,000 r.p.m. at 4 °C for 5 min. Serum was obtained by collecting the supernatant and stored at −80 °C until used for radioimmuno assay. Blood was sampled 2, 15 and 90 min after start of a 20 min restraint stress and Plexiglas tube under white light, and 1 h after stress. Plasma immunoreactive corticosterone titres were quantified using a kit according to the manufacturer’s recommendations (Corticosterone Elisa kit, AssayPro). Serum samples were diluted 1:100 prior to analysis, and data were analyzed by sigmoidal 4-parameter curve fit using Prism 6 (Graphpad). The minimal detectable dose for this assay is ~40 pg ml −1 , and intra- and inter-assay coefficients of variation are ~5% and 7%, respectively. Drug administration The histone acetyl-transferase inhibitor C646 (ref. 49 ; 4.45 μg kg −1 ) and the methyl-transferase inhibitor 3-deazaneplanocin A (ref. 50 ; 2 mg kg −1 ) in 0.9% saline were injected intraperitoneally (i.p.). Corticosterone (10 mg kg −1 , Sigma) in 3% EtOH (in 0.9% saline) and spironolactone (25 mg kg −1 , Sigma, previously reported to effectively block MR activity [51] ) in 3% EtOH were injected i.p. daily for 7 days. Control females received the same volume (10 μl g −1 ) of 0.9% saline or 3% EtOH. Twenty-four hours after injection, the animals were behaviourally tested or killed to extract the hippocampus for molecular analyses. Quantitative RT–PCR DNaseI-treated RNA (Allprep RNA/DNA kit; Qiagen) was reverse transcribed using the SuperScript First-Strand Synthesis System II for RT–PCR (Invitrogen, Carlsbad, CA, USA). Quantitative RT–PCR was performed in an ABI 7500 thermal cycler using TaqMan probes targeting only exons common to the different splice variants ( MR : Mm01241596_m1_m1, GR : Mm00433832_m1, Applied Biosystems Foster City, CA, USA). Western blotting Western blotting was conducted as previously described [25] . Briefly, 40 μg proteins from whole-cell extracts were resolved on 4–12% gradient SDS–PAGE and transferred onto a nitrocellulose membrane (Bio-Rad). Membranes were blocked in 5% milk then incubated in primary and secondary antibodies. MR polyclonal primary antibody produced in rabbits was applied at a concentration of 1:200 (MCR (H-300): sc-11412, Santa Cruz). GAPDH (1:1,000; rabbit monoclonal antibody; 14C10—#2118, Cell Signaling) was used as internal control. Each primary antibody was run on a separate day. Membranes were washed and incubated with secondary goat anti-rabbit antibody (IRDye 800 nm, 1:10,000; Li-Cor Biosciences). Band intensity was determined using an Odyssey IR scanner (Li-Cor Biosciences) and quantified with ImageJ. Samples from different groups were processed on the same blot. Bisulphite pyrosequencing Genomic DNA from hippocampus and sperm was extracted with Allprep kits (Qiagen) according to the manufacturer’s instructions. Bisulphite pyrosequencing was performed by EpigenDx, Inc., USA. Universally methylated and unmethylated DNA samples (Millipore Bioscience Research Regents) were used as controls. Chromatin immunoprecipitation ChIP was performed as described previously [25] using anti-acetyl-histone H4 (Lys5) (H4K5ac, Millipore, ChIPAb), anti-acetyl-histone H3 (Lys14) (H3K14ac, Millipore, ChIPAb), anti-trimethyl-histone H3 (Lys36) (H3K36me3, Millipore), anti-dimethyl-histone H3 (Lys4) (H3K4me2, Millipore), anti-dimethyl-histone H3 (Lys9) (H3K9me2, Millipore), anti-dimethyl-histone H3 (Lys27) (H3K27me2, Millipore) or mouse immunoglobulin-G (Millipore, 12–371B). DNA was quantified in immunoprecipitated samples by quantitative PCR in an Applied Biosystems 7500 Thermal Cycler using specific primers ( MR : forward, 5′-AACTGGGGGCTCAGAGATTT-3′; reverse, 5′-GCTCTTCCCAGGACTGACTG-3′. GR : forward, 5′-GCCCCTCTGCTAGAGTGACA-3′; reverse: 5′-GGAGGGAAAGCGAGTTTCTTM-3′; NFκB: forward: 5′-GCGCTGTGGCTGAAATAA-3′; reverse: 5′-TCATCTGCTTGTTCCCTCCT-3′; cFos: forward: 5′-TACGACCCCTTCAGGCATAC-3′; reverse: 5′-TAAAGGACGGCAGCACCTAC-3′; CREB: forward: 5′-AGGGAGGACGGTACCCAGTA-3′; reverse: 5′-TTCTTTGCTGGGAAGAAAGC-3′, Sox17: forward: 5′-CCACTCACTCTGAGGCTCGCTGTAG-3′; reverse: 5′-CCAAAGCAGACCTGAGGCTCGAA-3′, GAPDH: forward: 5′-CTCTGCTCCTCCCTGTTCC-3′ reverse: 5′-TCCCTAGACCCGTACAGTGC-3′) and SYBR green Mastermix (Qiagen) with the following cycling conditions: 10 min at 94 °C, 50 cycles of 20 s at 94 °C+1 min at 60 °C. Data were collected in the linear amplification range and each PCR experiment was repeated at least twice. Real-time quantitative RT–PCR was performed for every immunoprecipitated sample, immunoglobulin-G and input control and samples were run in triplicates. GAPDH was used as control gene. The relative proportion of immunoprecipitated fragments was determined based on the threshold cycle value ( C t) for each PCR reaction. The following equation was used for normalization: Fold difference versus negative control=2 −[( C t histone PTM/Ct input control)—( C t negative control/Ct input control)] . Statistical analyses Statistical analyses were performed using SPSS. EPM behavioural data were analyzed using two-tailed t -test. DRL and IntelliCages experiments were analyzed using repeated measurements analysis of variance with group (MSUS, control) as between subjects factor, and sessions or bins of sessions as within subject factors. Molecular experiments were analyzed by two-tailed t -test. Outliers with a mean value away from the group mean by ±2 s.d. were excluded. Significance was set at 0.05. Sample size was not predetermined with a statistical method but was similar to that reported in our previous publications on the MSUS model [13] , [40] , [41] , [42] . How to cite this article: Gapp, K. et al. Early life stress in fathers improves behavioural flexibility in their offspring. Nat. Commun. 5:5466 doi: 10.1038/ncomms6466 (2014).